No extension of quantum theory can have improved predictive power According to quantum theory, measurements generate random outcomes, in stark contrast with classical mechanics. This raises the question of whether there could exist an extension of the theory that removes this indeterminism, as suspected by Einstein, Podolsky and Rosen. Although this has been shown to be impossible, existing results do not imply that the current theory is maximally informative. Here we ask the more general question of whether any improved predictions can be achieved by any extension of quantum theory. Under the assumption that measurements can be chosen freely, we answer this question in the negative: no extension of quantum theory can give more information about the outcomes of future measurements than quantum theory itself. Our result has significance for the foundations of quantum mechanics, as well as applications to tasks that exploit the inherent randomness in quantum theory, such as quantum cryptography. Given a system and a set of initial conditions, classical mechanics allows us to calculate the future evolution to arbitrary precision. Any uncertainty we might have at a given time is caused by a lack of knowledge about the configuration. In quantum theory, on the other hand, certain properties—for example, position and momentum—cannot both be known precisely. Furthermore, if a quantity without a defined value is measured, quantum theory prescribes only the probabilities with which the various outcomes occur, and is silent about the outcomes themselves. This raises the important question of whether the outcomes could be better predicted within a theory beyond quantum mechanics [1] . An intuitive step towards its answer is to consider appending local hidden variables to the theory [2] . These are classical variables that allow us to determine the experimental outcomes (see later for a precise definition). Here we ask a new, more general question: is there any extension of quantum theory (not necessarily taking the form of hidden variables) that would convey any additional information about the outcomes of future measurements? We proceed by giving an illustrative example. Consider a particle heading towards a measurement device that has a number of possible settings, denoted by a parameter, A , corresponding to the different measurements that can be chosen by the experimenter. The measurement generates a result, denoted X . For concreteness, one could imagine a spin-1/2 particle incident on a Stern–Gerlach apparatus. Each choice of measurement corresponds to a particular orientation of the device, and the outcome is assigned depending on which way the beam is deflected. Within quantum theory, a description of the quantum state of the particle and of the measurement apparatus allows us to calculate the distribution, P X | A , of the outcome, X , for each measurement choice, A . 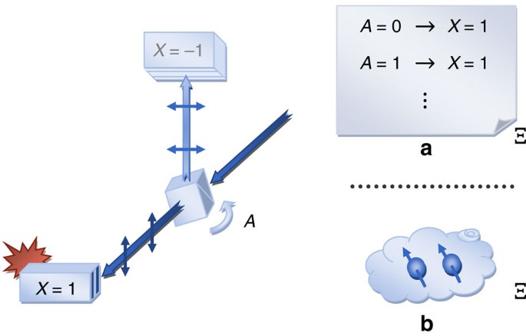Figure 1: Illustration of the scenario. A measurement is carried out on a particle, depicted as a photon measured using an arrangement comprising a polarizing beam splitter and two detectors. The measurement choice (the angle of the polarizing beam splitter) is denotedAand the outcome,X, is assigned −1 or 1 depending on which detector fires. On the right, we represent the additional information that may be provided by an extended theory, Ξ, shown here taking the form of either (a) hidden variables, that is, a classical list assigning outcomes, or (b) a more general (for example, quantum) system. Another example is described in Figure 1 . Figure 1: Illustration of the scenario. A measurement is carried out on a particle, depicted as a photon measured using an arrangement comprising a polarizing beam splitter and two detectors. The measurement choice (the angle of the polarizing beam splitter) is denoted A and the outcome, X , is assigned −1 or 1 depending on which detector fires. On the right, we represent the additional information that may be provided by an extended theory, Ξ, shown here taking the form of either ( a ) hidden variables, that is, a classical list assigning outcomes, or ( b ) a more general (for example, quantum) system. Full size image In this work, we consider the possibility that there exists further, yet to be discovered, information that allows the outcome X to be better predicted. We do not place any restrictions on how this information is manifest, nor do we demand that it allows the outcomes to be calculated precisely. In particular, it could be that the additional information gives rise to a more accurate distribution over the outcomes. For example, in an experiment for which quantum theory predicts a uniform distribution over the outcomes, X , there could be extra information that allows us to calculate a value, X ′, such that X = X ′ with probability 3/4 (in the model proposed by Leggett [3] , for instance, the local hidden variables provide information of this type). More generally, we allow for the possibility of an extended theory that provides non-classical information. For example, it could comprise a 'hidden quantum system', which, if measured in the correct way, gives a value correlated to X . Assumptions To formulate our main claim about the non-extendibility of quantum theory, we introduce a framework within which any arbitrary extra information provided by an extension of the current theory can be considered. In the following, we explain this framework on an informal level (see Supplementary Methods for a formal treatment). The crucial feature of our approach is that it is operational, in the sense that we only refer to directly observable objects (such as the outcome of an experiment), but do not assume anything about the underlying structure of the theory. Note that the outcome, X , of a measurement is usually observed at a certain point in spacetime. The coordinates of this point (with respect to a fixed reference system) can be determined operationally using clocks and measuring rods. Analogously, the measurement setting A needs to be available at a certain spacetime point (before the start of the experiment). To model this, we introduce the notion of a spacetime random variable (SV), which is simply a random variable together with spacetime coordinates ( t , r 1 , r 2 , r 3 ). Operationally, a SV can be interpreted as a value that is accessible at a given spacetime point ( t , r 1 , r 2 , r 3 ). We now model a measurement process as one that takes an input, A , to an output, X , where both X and A are SVs. Our result is based on the assumption that measurement settings can be chosen freely (which we call assumption FR ). We note that this assumption is common in physics, but often only made implicitly. It is, for example, a crucial ingredient in Bell's theorem (see ref. 4 ). Formulated in our framework, assumption FR is that the input, A , of a measurement process can be chosen such that it is uncorrelated with certain other SVs, namely all those whose coordinates lie outside the future lightcone of the coordinates of A . We note that this reference to a lightcone is only used to identify a set of SVs and does not involve any assumptions about relativity theory (see the Supplementary Information ). However, the motivation for assumption FR is that, when interpreted within the usual relativistic spacetime structure, it is equivalent to demanding that A can be chosen such that it is uncorrelated with any pre-existing values in any reference frame. That said, the lack of correlation between the relevant SVs could be justified in other ways, for example, by using a notion of 'effective freedom' (discussed in ref. 4 ). We also remark that Assumption FR is consistent with a notion of relativistic causality in which an event B cannot be the cause of A if there exists a reference frame in which A occurs before B . In fact, our criterion for A to be a free choice is satisfied whenever anything correlated to A could potentially have been caused by A . However, in an alternative world with a universal (frame-independent) time, one might reject assumption FR and replace it with something weaker, for example, that A is free, if it is uncorrelated with anything in the past with respect to this universal time. Nevertheless, since experimental observations indicate the existence of relativistic spacetime, we use a notion of free choice consistent with this. We additionally assume that the present quantum theory is correct (we call this assumption QM ). This assumption is natural because we are asking whether quantum theory can be extended. In fact, we only require that two specific aspects of quantum theory hold, and so split assumption QM into two parts. On an informal level, the first is that measurement outcomes obey quantum statistics, and the second is that all processes within quantum theory can be considered as unitary evolutions, if one takes into account the environment (see the Supplementary Information for more details). We remark that the second part of this assumption need only hold for microscopic processes on short timescales and does not preclude subsequent wavefunction collapse. Main findings Consider a measurement that depends on a setting A and produces an output X . According to quantum theory, we can associate a quantum state and measurement operators with this process from which we can compute the distribution P X | A . We ask whether there could exist an extension of quantum theory that provides us with further information (which we denote by Ξ) that is useful to predict the outcome. To keep the description of the information, Ξ, as general as possible, we do not assume that it is encoded in a classical system, but, instead, characterize it by how it behaves when observed. (Formally, we model access to Ξ analogously to the measurement of a quantum system, that is, as a process which takes an input SV and produces an output SV). We demand that Ξ can be accessed at any time (similarly to classical or quantum information held in a storage device) and that it is static, that is, its behaviour does not depend on where or when it is observed. Our main result is that we answer the above question in the negative, that is, we show that, using assumptions FR and QM , the distribution P X | A is the most accurate description of the outcomes. More precisely, for any fixed (pure) state of the system, the chosen measurement setting, A , is the only non-trivial information about X , and any extra information, Ξ, provided by an extended theory is irrelevant. We express this through the Markov chain condition This condition expresses mathematically that the distribution of X given A and Ξ is the same as the distribution of X given only A [5] . Hence, access to Ξ does not decrease our uncertainty about X , and there is no better way to predict measurement outcomes than by using quantum theory. In the Methods, we sketch the proof of this (the full proof is deferred to the Supplementary Information ). We now discuss experimental aspects related to our result. Note that at the formal level, we present a theorem about certain defined concepts on the basis of certain assumptions, hence what remains is to connect our definitions to observations in the real world, and experimentally confirm the assumptions, where possible. Assumption FR refers to the ability to make free choices and—while we can never rule out that the universe is deterministic and that free will is an illusion—this is in principle falsifiable, for example, by a device capable of guessing an experimentalist's choices before they are made. (See also ref. 6 where the possibility of weakening this assumption is discussed.) The validity of assumption QM could be argued for on the basis of experimental tests of quantum theory. However, the existence of the particular correlations we use in the second part of our proof is quantum-theory independent, so worth establishing separately. Because of experimental inefficiencies, these correlations cannot be verified to arbitrary precision. 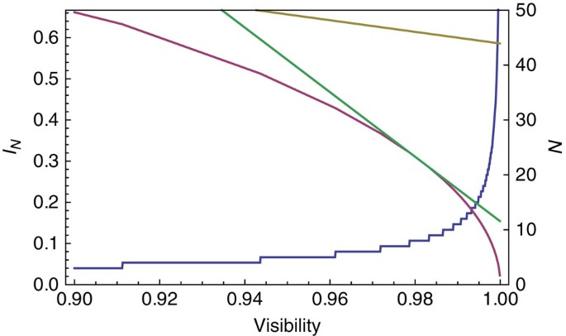Figure 2: Achievable values ofINdepending on the experimental visibility. This figure relates to the measurement setup used for testing the accuracy of assumptionQMas described in the Methods. The setup involves two parties and is parameterized by the number of possible measurement choices available to each party,N. The plot gives the minimumINachievable depending on the visibility (red line), which determines the smallest upper bound on the variational distance from the perfect Markov chain condition (1) that could be obtained with that visibility (see equation (8)). It also shows the optimal value ofNwhich achieves this (blue line). For comparison, the values achievable usingN=2, which corresponds to the CHSH measurements26(yellow line), and the caseN=8, which is optimal for visibility 0.98 (green line), are shown. Figure 2 bounds our ability to experimentally establish (1) depending on the quality of the setup used (characterized here by the visibility). For more details, see the Methods. Figure 2: Achievable values of I N depending on the experimental visibility. This figure relates to the measurement setup used for testing the accuracy of assumption QM as described in the Methods. The setup involves two parties and is parameterized by the number of possible measurement choices available to each party, N . The plot gives the minimum I N achievable depending on the visibility (red line), which determines the smallest upper bound on the variational distance from the perfect Markov chain condition (1) that could be obtained with that visibility (see equation (8)). It also shows the optimal value of N which achieves this (blue line). For comparison, the values achievable using N =2, which corresponds to the CHSH measurements [26] (yellow line), and the case N =8, which is optimal for visibility 0.98 (green line), are shown. Full size image We proceed by discussing previous work on extensions of quantum theory. To the best of our knowledge, all such extensions that have been excluded to date can also be excluded using our result. The question asked by Einstein, Podolsky and Rosen [1] was whether quantum mechanics could be considered complete. They appealed to intuition to argue that an extended theory should exist and one might then have hoped for a deterministic completion, that is, one that would uniquely determine the measurement outcomes—contrast this with our (more general) notion, where the extended theory may only give partial information. Bell [2] famously showed that a deterministic completion is not possible when the theory is supplemented by local hidden variables. (To relate this back to our result, this corresponds to the special case where the further information, Ξ, is a classical value specified by the local hidden variables. A short discussion on the term 'local' can be found in the Supplementary Information .) Recently, a conclusion [7] similar to Bell's has been reached using the Kochen–Specker theorem [8] . These results have been extended to arbitrary (that is, not necessarily local) hidden variables [9] , [10] , under the assumption of relativistic covariance (see also ref. 11 , as well as ref. 12 , where a condition slightly weaker than locality is used to derive a theorem similar to Bell's). The aforementioned papers left open the question of whether there could exist an extended theory that provides further information about the outcomes without determining them completely. (Note that, in his later works, Bell uses definitions that potentially allow probabilistic models [13] . However, as explained in the Supplementary Information , non-deterministic models are not compatible with Bell's other assumptions.) In the case that the further information takes the form of local hidden variables, an answer to the above question can be found in refs 3 , 14 , 15 , and the strongest result is that any local hidden variables are necessarily uncorrelated with the outcomes of measurements on Bell states [15] . (We remark that the model in ref. 3 also included non-local hidden variables. However, we have not referred to these in this paragraph, because, as mentioned below in the context of de Broglie–Bohm theory, the presence of non-local hidden variables contradicts assumption FR ). In the present work, we have taken this idea further and excluded the possibility that any extension of quantum theory (not necessarily in the form of local hidden variables) can help predict the outcomes of any measurement on any quantum state. In this sense, we show the following: under the assumption that measurement settings can be chosen freely, quantum theory really is complete. We remark that several other attempts to extend quantum theory have been presented in the literature, the de Broglie–Bohm theory [16] , [17] being a prominent example (this model recreates the quantum correlations in a deterministic way but uses non-local hidden variables, see ref. 18 for a summary). Our result implies that such theories necessarily come at the expense of violating assumption FR . Another way to generate candidate extended theories is via models that simulate quantum correlations. We discuss the implications of our result in light of such models in the Supplementary Information . In addition, we remark that a claim in the same spirit as ours has recently been obtained on the basis of the assumption of non-contextuality [19] . Randomness is central to quantum theory, and with it comes a range of philosophical implications. In this article, we have shown that the randomness is inherent: any attempt to better explain the outcomes of quantum measurements is destined to fail. Not only is the universe not deterministic, but quantum theory provides the ultimate bound on how unpredictable it is. Aside from these fundamental implications, there are also practical ones. In quantum cryptography, for example, the unpredictability of measurement outcomes can be quantified and used to restrict the knowledge of an adversary. Most security proofs implicitly assume that quantum theory cannot be extended (although there are exceptions, the first of which was given in ref. 20 ). However, in this work, we show that this follows, if the theory is correct. Sketch of the proof Our main result is the following theorem whose proof we sketch here (see the Supplementary Information for the formal treatment). Theorem 1 : For any quantum measurement with input SV A and output SV X and for any additional information, Ξ, under assumptions QM and FR , the Markov chain condition (1) holds. The proof is divided into three parts. The first two are related to a Bell-type setting, involving measurements on a maximally entangled state. In Part I, we show that assumption FR necessarily enforces that Ξ is non-signalling (in the sense defined below). In Part II, we show that for a particular set of bipartite correlations, if Ξ is non-signalling, it cannot be of use to predict the outcomes. These correlations occur in quantum theory (cf. the first part of assumption QM ) when measuring a maximally entangled state, and hence we conclude that no Ξ can help predict the outcomes of measurements on one-half of such a state. Finally, in Part III, we use the second part of assumption QM to argue that this conclusion also applies to all measurements on an arbitrary (pure) quantum state. Together, these establish our claim. The bipartite scenario used for the first two parts of the proof involves two quantum measurements, with inputs A and B and respective outputs X and Y . The setup is such that the two measurements are spacelike separated in the sense that the coordinates of A are spacelike separated with the coordinates of Y , and, likewise, those of B are spacelike separated with those of X . As mentioned in the main text, we model the information provided by the extended theory, Ξ, by its behaviour under observation. We introduce a SV, C , which can be thought of as the choice of what to observe, and another SV, Z , which represents the outcome of this observation (all the SVs used in the setup are shown in Supplementary Fig. S1 ). In terms of these variables, our main result, equation (1), can be restated that for all values of a , c and x , we have (Note that we use lower case to denote specific values of the corresponding upper case SVs). Proof part I The entire setup described above (including the extra information Ξ, accessed by choosing an observable, C , and obtaining an outcome, Z ) gives rise to a joint distribution P XYZ | ABC . The purpose of this part of the proof is to show that assumption FR implies that P XYZ | ABC must satisfy particular constraints, called non-signalling constraints, which characterize situations where operations on different isolated systems cannot affect each other. Formally, these are We remark that the observation that the assumption of free choice gives rise to certain non-signalling constraints has been made already in ref. 11 , and a similar argument has been presented by Gisin [9] and Blood [10] . (Note that the arguments in refs 9 , 10 implicitly assume that measurements can be chosen freely). Assumption FR allows us to make A a free choice and hence we have (the setup is such that the measurements specified by A and B are spacelike separated and, furthermore, Ξ is static; so, we can consider the case where its observation is also spacelike separated from the measurements specified by A and B ). Furthermore, using the definition of conditional probability , we can write where we inserted (6) to obtain the second equality. Similarly, we have Comparing these two expressions for P YZA | BC yields the desired non-signalling condition (3). By a similar argument, the other non-signalling conditions can be inferred from assumption FR . Proof part II For the second part of the proof, we consider the distribution P XY | AB resulting from certain appropriately chosen measurements on a maximally entangled state. We show that any enlargement of this distribution (through a system Ξ that is accessed in a process with input SV C and output SV Z ) to a distribution P XYZ | ABC that satisfies the above non-signalling conditions is necessarily trivial in the sense that Ξ is uncorrelated to the rest. For this, we draw on ideas from non-signalling cryptography [20] , which are related to the idea of basing security on the violation of Bell inequalities [21] . Technically, we employ a lemma (see Lemma 1 in the Supplementary Information ), whose proof is based on chained Bell inequalities [22] , [23] and generalizes results of refs 15 , 24 . Consider any bipartite measurement with inputs A ∈ {0, 2..., 2 N −2} and B ∈ {1, 3..., 2 N −1}, for some positive integer N , and binary outcomes, X and Y . The correlations of the outcomes can be quantified by Our lemma then asserts that, under the non-signalling conditions derived in Part I, for all a , b , c and x , where D is the variational distance, defined by The variational distance has the following operational interpretation: if two distributions have variational distance at most δ , then the probability that we ever notice a difference between them is at most δ . The argument up to here is formally independent of quantum theory. However, as we describe below (see the Experimental verification section), for any fixed orthogonal rank-one measurement on a two-level subsystem, one can construct 2 N −1 other measurements such that, according to quantum theory, applying these measurements to maximally entangled states leads to correlations that satisfy . It follows that, in the limit of large N , an arbitrarily small bound on D ( P Z | abcx , P Z | abc ) can be obtained. We thus conclude that P Z | abcx = P Z | abc , which, by the non-signalling condition (4), also implies (2). We have therefore shown that the relation (1) holds for the outcome X of any orthogonal rank-one measurement on a system that is maximally entangled with another one (our claim can be readily extended to systems of dimension 2 t for positive integer t by applying the result to t two-level systems). We also remark that Markov chains are reversible, that is, P Z | abcx = P Z | abc implies P X | abcz = P X | abc , which together with the non-signalling conditions gives P X | abcz = P X | a . This establishes that, for any choices of B and C , learning Z does not allow an improvement on the quantum predictions, P X | a . Proof part III To complete our claim, it remains to show that the Markov chain condition (1) holds for measurements on arbitrary states (not only for those on one part of a maximally entangled state shared between two sites). The proof of this proceeds in two steps. The first is to append an extra measurement with outcome X ′, chosen such that the pair ( X , X ′) is uniformly distributed. In the second step, we split the measurement into two conceptually distinct parts, where, in the first, the measurement apparatus becomes entangled with the system to be measured (and, possibly the environment) and, in the second, this entangled state is measured giving outcomes ( X , X ′). As these outcomes are uniformly distributed, the state before the measurement can be considered maximally entangled, so that (1) holds with X replaced by ( X , X ′). This implies (1) and hence completes the proof of Theorem 1. Experimental verification As explained above, the validity of parts of assumption QM can be established by a direct experiment. In particular, to verify the existence of the correlations required for Part II of the proof, that is, those with small I N , one should generate a large number (much larger than N ) of maximally entangled particles and distribute them between the measurement devices. At spacelike separation, a two-level subsystem (for example, a spin degree of freedom) should then be measured, the measurement being picked at random from those specified below, and the results recorded. This is repeated for all of the particles. The measurement choices and results are then collected and used to estimate the terms in I N using standard statistical techniques. For an arbitrary orthogonal basis {|0〉,|1〉}, the required measurements can be constructed in the following way. Recall that the choice of measurement on one side takes values A ∈ {0, 2..., 2 N −2} and similarly, B ∈ {1, 3..., 2 N −1}. We define a set of angles and states The required measurement operators are then and Although quantum theory predicts that arbitrarily small values of I N can be obtained for large N , due to imperfections and errors in the devices, it will not be possible to experimentally achieve this. In ref. 25 , a discussion of the achievable values of I N with imperfect visibilities was given. For visibilities less than 1, it is not optimal to take N as large as possible to minimize the observed I N . Thus, to get increasingly small bounds on the variational distance in (8), one must increase the experimentally obtained visibilities as well as the number of measurement settings (see Fig. 2 ). How to cite this article: Colbeck, R. & Renner, R. No extension of quantum theory can have improved predictive power. Nat. Commun. 2:411 doi: 10.1038/ncomms1416 (2011).